Attosecond nonlinear optics using gigawatt-scale isolated attosecond pulses High-energy isolated attosecond pulses required for the most intriguing nonlinear attosecond experiments as well as for attosecond-pump/attosecond-probe spectroscopy are still lacking at present. Here we propose and demonstrate a robust generation method of intense isolated attosecond pulses, which enable us to perform a nonlinear attosecond optics experiment. By combining a two-colour field synthesis and an energy-scaling method of high-order harmonic generation, the maximum pulse energy of the isolated attosecond pulse reaches as high as 1.3 μJ. The generated pulse with a duration of 500 as, as characterized by a nonlinear autocorrelation measurement, is the shortest and highest-energy pulse ever with the ability to induce nonlinear phenomena. The peak power of our tabletop light source reaches 2.6 GW, which even surpasses that of an extreme-ultraviolet free-electron laser. Attosecond science has emerged as an important research area of ultrafast phenomena within the past decade [1] . Owing to its numerous successes, attosecond science has created important new knowledge (see review ref. 2 ) of the fundamental science of the interaction between electrons and photons. Recently, some key research topics have been identified, which are expected to make major breakthroughs for the next attosecond frontiers, such as the MHz high-repetition high-order harmonic (HH) frequency combs for the joint frontier of precision spectroscopy and ultrafast science, attosecond-pump/attosecond-probe experiments for observing and controlling electronic processes in atomic and molecular physics, and nonlinear science occurring on the attosecond time scale. To seriously tackle the above interesting research topics, one of the most important issues is the development of high-power isolated attosecond pulses (IAPs) and/or attosecond pulse trains. IAPs and attosecond pulse trains are produced using HH generation (HHG) [3] , [4] in gases. To date, high-power attosecond pulse trains have successfully been generated owing to research on HH energy scaling using a loose-focusing geometry [5] . Attosecond pulse trains with sufficiently high energy in the microjoule range with a high conversion efficiency on the 10 −4 level were generated [6] , which are intense enough for implementing some applications, such as nonlinear attosecond optics [7] , [8] without the assistance of laser pulses, single-shot femtosecond holography [9] and an external injector for a seeded [10] free-electron laser (FEL) in the extreme-ultraviolet (XUV) region. In contrast, the output energy of IAPs is still not sufficient for various applications, although the shortest pulse duration achieved is sub-100 as in ref. 11 . The widespread application of IAPs has been limited because of the low photon flux and the complexity of the laser systems required to produce IAPs (see review in ref. 12 ). At present, the highest IAP energy is less than a few tens of nanojoules [13] at a 27-eV photon energy. The highest conversion efficiency demonstrated is only 10 −5 to 10 −6 , even if Xe gas is used. Consequently, the production, characterization and application of high-energy IAPs are still under active investigation. Here we report a harmonic generation method suitable for nonlinear pump/probe experiments that demonstrates the capability of time-resolving attosecond dynamical processes with IAPs. Our generation scheme is robust and straightforward for scaling up the HH energy, which is based on an infrared two-colour (TC) laser field synthesis [14] and the energy-scaling method [5] . By carefully designing the HHG configuration, we can obtain IAPs with a record energy of up to 1.3 μJ at ~30 eV, thus demonstrating a >100-fold energy enhancement compared with previous reports [13] . The conversion efficiency achieved is improved to 1.1 × 10 −4 , owing to favourable phase-matching technique. Even though our TC method leads to weak multiple burst emissions [14] occurring for specific combinations of the carrier-envelope phase (CEP) and relative phase, we nevertheless can observe the nonlinear signal corresponding to IAPs, because the nonlinear process automatically selects predominantly the contributions from the most intense IAPs generated for certain favourable phase combinations. In fact, we present the direct temporal characterization of an IAP by a second-order autocorrelation (AC) measurement using nonlinear phenomena in N 2 molecules. The AC measurement is one of the simplest applications of a nonlinear pump/probe experiment. The measured AC traces indicate not only the temporal duration of the interacting IAPs but also provide evidence for the nonlinear interaction with the target medium. From the 500-as pulse duration determined by the AC measurement, the IAP’s peak power can be evaluated to be 2.6 GW with weak satellite pulses at the generation point. Furthermore, in our TC-HHG experiment, we create a mid-plateau region exhibiting a quasi-continuous spectrum with an energy of 10 μJ. From the AC measurement of this quasi-continuous spectrum at the mid-plateau, we evaluate that a quasi-IAP with pulse duration of 375 as with ~0.27 intensity satellite pulses at ±6.7 fs dominated the nonlinear interaction with the N 2 target. Harmonic spectra and output energy We strictly considered and designed the configuration of a thoroughly engineered generation scheme (see Methods section) for scaling up the HH output energy. 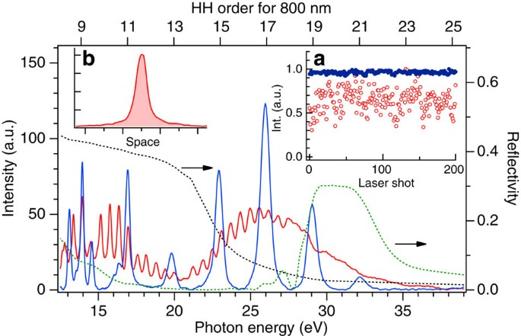Figure 1: Experimentally obtained single-shot HH spectra from Xe. Blue curve: OC laser field (800 nm: 11 mJ); red curve: TC laser field (800 nm: 9 mJ+1,300 nm: 2.5 mJ). Green dotted curve: reflectivity of the Sc/Si multilayer mirror; black dotted curve: reflectivity of the SiC bulk mirror. Inset: (a) measured intensity variation of the HH cutoff (~29 eV: 19th HH order) over 200 laser shots. (b) The spatial profile of the cutoff harmonics of the TC-HHG. Figure 1 shows typical single-shot HH spectra of Xe gas as function of photon energy. The focused intensity in the TC case ( I TC ) was ~5 × 10 13 W cm −2 with an intensity ratio of ξ ~0.15. The HH yield is optimized by adjusting the focusing point with respect to the gas cell and by varying the gas pressure. As the difference between the dispersions for the 800- and 1,300-nm pulses in Xe is negligible, the phase-matching condition can be satisfied by optimizing the gas pressure. The HH yield gradually increases as the Xe gas pressure increases, and exhibits a quadratic dependence on pressure. This means the conversion efficiency and the photon flux of HHG depend on the Xe gas pressure. The cutoff intensity of TC-HHG is optimized at a gas pressure of ~0.8 Torr, which is in good agreement with the optimum gas pressure predicted by the phase-matching theory [15] under these experimental conditions. Figure 1: Experimentally obtained single-shot HH spectra from Xe. Blue curve: OC laser field (800 nm: 11 mJ); red curve: TC laser field (800 nm: 9 mJ+1,300 nm: 2.5 mJ). Green dotted curve: reflectivity of the Sc/Si multilayer mirror; black dotted curve: reflectivity of the SiC bulk mirror. Inset: ( a ) measured intensity variation of the HH cutoff (~29 eV: 19th HH order) over 200 laser shots. ( b ) The spatial profile of the cutoff harmonics of the TC-HHG. Full size image When the one-colour (OC) field is focused to an intensity of 7 × 10 13 W cm −2 , the HH spectrum has a discrete structure (blue curve). In the TC scheme (red curve), a quasi-continuous HH spectrum appears in the lower-order region, whereas the quasi-continuous HH disappears at harmonic orders higher than the 17th. We can clearly see a smooth continuum HH spectrum around the HH cutoff region. Note that the intensity of the TC-HH is comparable to that of the OC-HH. From the wavelength-scaling law of the TC-HHG (see Fig. 8) under the ξ =0.15 condition, the conversion efficiency decreases only by a factor of (1,300/800) −0.7 ~0.71 compared with the OC-HHG case. The maximum HH photon energy is slightly extended to 35 eV even though the focused intensity is lower than for the OC-HHG. This photon energy extension is explained by the cutoff formula for TC-HHG [14] . The inset (a) of Fig. 1 shows the measured intensity variation of the HH cutoff (~29 eV: 19th HH order) over 200 laser shots. The intensity of the OC-HH has a high stability, as shown by the blue points, whereas the intensity of the TC-HH (red points) fluctuates between 1 and 0.3. As already reported in ref. 14 , these variations are due to the intensity changes of the TC field caused by random fluctuations in the CEP value of the non-CEP-stabilized Ti:sapphire laser and slight jitter of the relative phase introduced by the Mach–Zehnder interferometer used for creating the TC fields. According to the discussion of the variations of these two kinds of phase effects (see Discussion section), the HH yield at the cutoff should be maximized, when the continuous spectrum frequently appears for certain ‘good’ combinations of the CEP and relative phase, whereas only weak HH exhibiting the quasi-continuum spectrum is generated for ‘bad’ phase combinations. We have actually observed this correlation between the HH yield and the spectral shape in the experiment. Note that harmonic shots with the quasi-continuum spectrum hardly contribute to form the AC trace, because their intensity is quite low. The output beam divergence of the TC-HH at the cutoff was measured to be ~0.5 mrad full-width half maximum with a Gaussian-like profile (see Fig. 1b inset). The almost perfect Gaussian profile of the HH suggests that there is no density disturbance due to high ionization in the harmonic medium. The pulse energy of the continuous HH spectrum (28–35 eV) is evaluated to be 1.3 μJ with a conversion efficiency of 1.1 × 10 −4 from the input TC energy (800 nm: 9 mJ+1,300 nm: 2.5 mJ). This value is almost 100-fold higher than the highest pulse energies ever reported before [13] . The generation efficiency from the Ti:sapphire laser is 3.7 × 10 −5 , because 30 mJ of Ti:sapphire energy was used for creating the TC field. Moreover, the mid-plateau region (14–29.5 eV) exhibiting a quasi-continuous spectrum in the TC-HHG has an output energy of ~10 μJ. Nonlinear AC measurement for attosecond pulses To evaluate the temporal characteristics of the microjoule HH fields, we utilized an AC method using a spatially split autocorrelator. We employed two concave mirrors ( R =200 mm) for focusing the HH: one is a bulk SiC mirror for the mid-plateau and the other is a Sc/Si multilayer mirror for the cutoff. The reflectivity for each concave mirror is shown in Fig. 1 . We have adopted the N + ion yield from fragmenting N 2 molecules as the indicator of the second-order AC signal (see Methods section). This choice is motivated by the findings of our earlier experiment [8] , in which the N + ion yield was sufficiently high to obtain the AC trace of an attosecond pulse in the relevant HH photon energy region. The dotted curves in the top panels of Fig. 2a,b are the measured AC traces of the mid-plateau TC-HH and OC-HH fields, respectively. The signals at each delay time are obtained by accumulating signals for 1 × 10 3 laser shots. We can see distinct peaks emerge at every half period (1.33 fs) of the Ti:sapphire laser field in the AC trace depicted in the top panel of Fig. 2b . This result ensures that our AC measurement can certainly reveal the temporal shape in the attosecond regime. In contrast, the four peaks corresponding to multiple bursts on both side of the main peak (0 fs) are well suppressed in the TC-HH, even though we can observe the side peaks at ~±6.7 fs (indicated by arrows in Fig. 2a ) with a relative AC amplitude of ~0.45 compared with the main peak. These two side peaks are consistent with our simulated result (see Discussion section) of the TC-HHG. 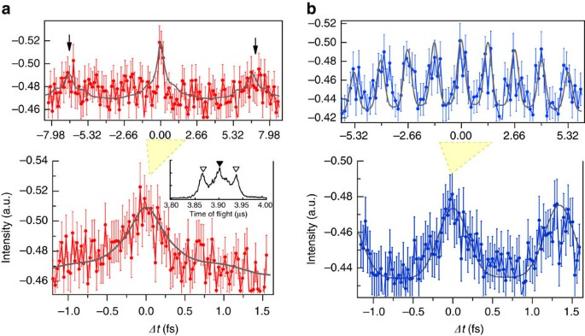Figure 2: Measured AC traces from the side peak of N+ion signals. (a) Mid-plateau of TC-HH; (b) mid-plateau of OC-HH. The time resolutions of the top and bottom panels correspond to 148 and 28 as, respectively. The error bars show the s.d. of each data point. The grey solid profiles are the AC traces of the simulated HH spectrum. Inset of (a): measured TOF spectrum of ions at aroundm/z=14. The inverted triangles and black-filled inverted triangle correspond to the KE of 3 and 0 eV, respectively. Figure 2: Measured AC traces from the side peak of N + ion signals. ( a ) Mid-plateau of TC-HH; ( b ) mid-plateau of OC-HH. The time resolutions of the top and bottom panels correspond to 148 and 28 as, respectively. The error bars show the s.d. of each data point. The grey solid profiles are the AC traces of the simulated HH spectrum. Inset of ( a ): measured TOF spectrum of ions at around m / z =14. The inverted triangles and black-filled inverted triangle correspond to the KE of 3 and 0 eV, respectively. Full size image To observe the pulse duration more precisely, we increased the time resolution of the AC measurement by reducing the delay step from 148 to 28 as. The bottom panels in Fig. 2 show the measured AC signal for OC-HH (blue points) and TC-HH (red points). In the mid-plateau of TC-HH, the full-width half maximum of the AC was measured to be τ AC =(530±75) as by fitting the trace with a Gaussian function (not shown). The pulse duration is thus τ HH = τ AC / ~375 as. On the other hand, the measured AC duration for the OC-HHG case was τ AC =(490±60) as. Thus, the duration of each peak in the attosecond pulse train is evaluated to be τ HH ~350 as, which is slightly shorter than the pulse duration of the TC-HH. The broadening of the AC duration of the TC-HH compared with the OC-HH case is owing to the fact that the AC trace of the TC-HH originates from the temporal profiles averaged over the random CEP and slightly fluctuating relative phase. In addition, the HH spectral shapes are different in both cases. As we successfully obtained the AC trace of the TC-HH in the mid-plateau, we furthermore explored the temporal characterization for the HH cutoff. In this experiment, we switched the focusing mirror from the SiC mirror to the Sc/Si multilayer mirror. The signal is scanned every 148 as from −8.5 to 8.5 fs with 1 × 10 3 laser shot accumulation at each delay point. The resultant signal points versus delay are shown in the top panel in Fig. 3 . Three distinct signal points around 0 delay seem to be a correlation peak and there are no noticeable side peaks in this figure, although our simulation result (see Discussion section) exhibits side peaks at ±6.7 fs with ~0.2 relative AC amplitude compared with the maximum peak at 0 delay. To confirm that the signal around 0 delay is certainly the correlation signal and that there are no significant side peaks at ±6.7 fs, we performed a high-resolution AC measurement in the delay scanning ranges around 0 fs and ±6.7 fs, as shown in the bottom panels in Fig. 3 . We accumulated 1 × 10 3 laser shots at each delay point and set the scanning delay step Δ t to be 28 as. We can demonstrate a clear peak at 0 delay as an AC in the middle-bottom panel in Fig. 3 . The AC duration was evaluated to be τ AC =(700±90) as by fitting the experimental trace to a Gaussian function; hence, the pulse duration is estimated to be τ HH ~500 as. We also find that there are no noticeable side peaks in the measured AC traces in the left-bottom and right-bottom panels in Fig. 3 . This is owing to the fact that the background noise amplitude (see Methods section) is comparable to the amplitude of the side peaks expected from our simulation. The noise magnitude against the peak AC amplitude is estimated to be ~0.24; thus, we cannot clearly find side peaks with amplitudes <0.24. In other words, we can safely conclude that the side-peak ratio should be <0.24. As discussed below, we can find both pre- and post-pulse in the calculated temporal profile at any CEP and relative phase. By assuming that the HH pulse consists of three (pre-, main and post-) pulses and the upper limit of the side peaks in the AC trace should be 0.24, we can estimate the possible largest peak height ratio of the pre- and post-pulses to be ~0.14. Further detailed analysis of the pre-/post-pulse issue is presented in the next section with the help of our numerical model of the TC-HH and statistical analysis of the relative phase. 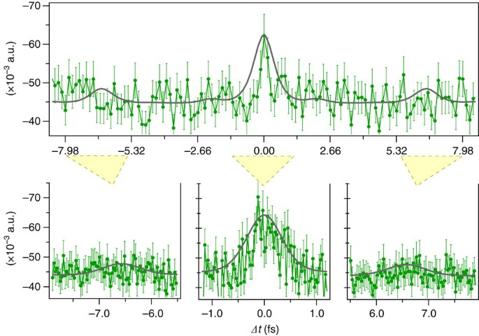Figure 3: Measured AC traces of an IAP obtained from the side peak of N+ion signals. The time resolutions of the top and bottom panels correspond to 148 and 28 as, respectively. The error bars show the s.d. of each data point. The grey solid profiles are AC traces obtained using the simulated HH fields. Figure 3: Measured AC traces of an IAP obtained from the side peak of N + ion signals. The time resolutions of the top and bottom panels correspond to 148 and 28 as, respectively. The error bars show the s.d. of each data point. The grey solid profiles are AC traces obtained using the simulated HH fields. Full size image From the measured pulse energy and pulse duration, the peak power of the IAP nonlinearly interacting with the target medium is evaluated to be 2.6 GW with weak satellite pulses (see Discussion section). This ultrahigh power from our tabletop light source even surpasses that from a compact XUV FEL [16] , [17] . The peak brightness is also estimated to be ~2 × 10 30 photons per s −1 mm −2 mrad −2 , assuming a 60-μm beam diameter at the exit of the gas cell. Finally, we examine attosecond pulse generation in our TC-HH scheme by numerical simulations. In these simulations, the single-atom response is calculated within the strong-field approximation. The propagation of the TC laser pulse and the high harmonics are computed separately in cylindrical coordinates [14] , [18] . All the parameters, such as laser intensity, target gas pressure and medium length, are determined by the experimental conditions. Here we assume that the CEP CE fluctuates randomly during the AC measurement, whereas the statistical fluctuations of the relative phase 0 are characterized by the measured histogram of the relative phase in the TC interferometer. To evaluate the relative phase variation with time in the TC interferometer, we injected a continuous-wave (CW) laser beam with a wavelength of 547 nm into the TC interferometer in this measurement. We recorded spatial interference fringes on the superposed beam profile of the CW laser with a charge-coupled device camera (exposure time: ~10 μs with 10 Hz repetition rate, which is synchronized with the pump laser) during ~35 min, which is equivalent to the data acquisition time of one AC trace in our measurements. The phase of the spatial fringes at each recorded profile was converted to the relative delay and relative phase corresponding to the 1,300-nm field. The measured time evolution of the relative phase, 0 , is shown in Fig. 4a . We can then evaluate the s.d. of 0 fluctuations, σ , to be 0.23 π from this measurement, whereas the offset of 0 is arbitrary. We adjust the offset in Fig. 4a such that the average of 0 is equal to 0. To improve the S/N ratio of the AC trace, we overlapped ten AC traces in Figs 2 and 3 . The σ -value with a typical normal distribution of the ten AC traces' 0 fluctuations was almost the same during the experiment, even though the phase profile as a function of time was different. 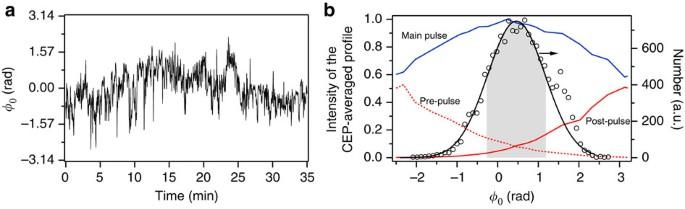Figure 4: Evaluation of the relative phase. (a) Measured relative phase versus time. (b) A histogram obtained fromawith a normal distribution fit (black solid curve). The intensity ratio of the CEP-averaged profile of the main (blue solid curve), pre- (red dotted curve) and post-pulse (red solid curve). The grey-filled area corresponds to the ±σarea. Figure 4: Evaluation of the relative phase. ( a ) Measured relative phase versus time. ( b ) A histogram obtained from a with a normal distribution fit (black solid curve). The intensity ratio of the CEP-averaged profile of the main (blue solid curve), pre- (red dotted curve) and post-pulse (red solid curve). The grey-filled area corresponds to the ± σ area. Full size image The histogram of our measured relative phase exhibits a typical normal distribution expressed by with a s.d., σ , of 0.23 π (see Fig. 4b ). The mean value of 0 , denoted as 0 in this equation, cannot be determined by our jitter measurement. Nevertheless, we set 0 to be 0.14 π rad in our averaging procedure in the calculations for reasons discussed below. Using the parameters mentioned above, we first calculate the temporal intensity profile for each 0 (calculation step: 100 mrad) value, varying CE in the range from − π /2 to π /2; later, we average the calculated HH intensity profile. We call the temporal profile of this averaged field the ‘CEP-averaged temporal profile’ at each 0 (see Fig. 5 ). Note that we adjust the offset of the time axis of each temporal profile of the HH field so as to locate the highest peak at the time origin before CEP averaging. This adjustment is consistent with the temporal profile to be measured with the spatially split AC technique, because the delay time (Δ t ) at the highest AC signal does not indicate the absolute time of the HH emission with respect to the driving TC-HH field, but coincides with the zero delay time between two replicas of the measured pulse. In an actual setup (see Fig. 9), we produce two time-delayed replica pulses from one HH pulse using two silicon beam splitters placed at Brewster’s angle for the driving field [19] . 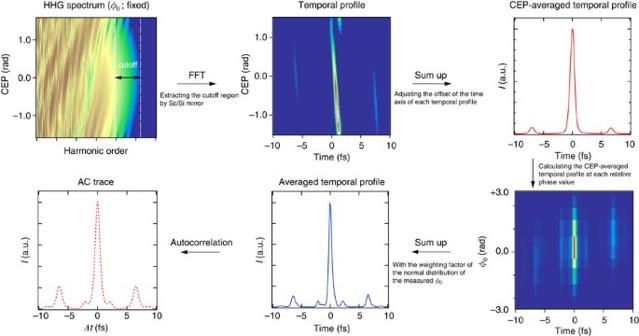Figure 5: Calculation procedure. Calculation procedure for evaluating the temporal profile of HHs. Figure 5: Calculation procedure. Calculation procedure for evaluating the temporal profile of HHs. Full size image After performing the CEP average, we superpose the ‘CEP-averaged temporal profiles’ at each 0 (see Fig. 5 ) with the above-mentioned weighting factor of the normal distribution of 0 (see solid black curve in Fig. 4b ). We have numerically searched for the mean value, 0 , in the normal distribution so as to minimize the side peaks of the superposed temporal profile, and then found 0 to be 0.14 π rad as mentioned above. This numerical procedure is compatible with our experimental approach of adjusting the relative phase in the TC interferometer such that the TC-HH exhibits the continuous spectrum most frequently. Thus, it is justified to set 0 to be 0.14 π rad in the normal distribution. The resulting 0 -weighted superposition of the ‘CEP-averaged temporal profile’, which we call the ‘averaged temporal profile’, in the mid-plateau region is shown as red-filled curve in Fig. 6a and that in the cutoff region is shown as green-filled curve in Fig. 6b . The averaged temporal profile includes both the effect of random fluctuation of CE and the measured relative phase jitter of 0 . The overall selected bandwidths of the mid-plateau and cutoff harmonics are 13–29 eV and 27–36 eV, which are determined by the reflectivity of the SiC and Sc/Si mirrors, respectively. Note that 13–23 eV HH effectively contribute to creating the temporal profile in the mid-plateau TC-HH profile due to the reflectivity edge of the SiC mirror. We notice that two satellite pulses appear at ±6.7 fs in both TC-HH profiles. The relative intensity of the higher satellite pulse compared with the main pulse for the mid-plateau TC-HH is 0.27. In contrast, the relative intensity of the cutoff TC-HH is considerably decreased to 0.1. Note that this side-peak intensity can be decreased by extracting slightly higher cutoff harmonic orders (>29 eV). We also observe a background pedestal under the main pulse in both TC-HH profiles. This small pedestal originates from weak multiburst emission around the centre of the TC electric field at the ‘wrong’ combinations of CEP and relative phase. The intensity of this pedestal is very low, because the HH yield is also low. Even though the temporal profile has side peaks (~0.27 relative intensity) at ±6.7 fs, the mid-plateau of TC-HH results in an IAP profile having a 390-as temporal duration for the central pulse. When we extract the cutoff harmonics, the expected temporal duration is 525 as with weak satellite pulses. We also calculated the AC trace by averaging over the CEP and relative phase according to the procedure shown in Fig. 5 , the simulated results are shown by dashed curves in Fig. 6 and solid curves in Figs 2 and 3 . As shown in these figures, the calculated AC traces are in good agreement with the experimental data. We can clearly find a significant reduction of the pulses forming an attosecond pulse train with a period of 1.33 fs in both TC-HH fields by comparing these profiles with that of the OC-HH in the mid-plateau region. Thus, we can conclude that the intensity of multiple burst emissions in our TC-HHG can be significantly reduced compared with another gating method [20] , [21] . In fact, the previously reported AC profile [21] exhibits a duration in the femtosecond region when a non-CEP-stabilized multicycle driving laser was utilized for generating IAPs. We notice that the intensity ratio between the main (0 fs) and the satellite pulses (±6.7 fs) of the AC traces is much higher (approximately twice) than that of the temporal profiles shown in Fig. 6 , respectively. As the temporal profile of the TC-HH cutoff is composed by three pulses, the simulated AC intensity ratio of the side peak is ~0.2 compared with the main pulse, even though the temporal intensity ratio of the side peak is ~0.1. 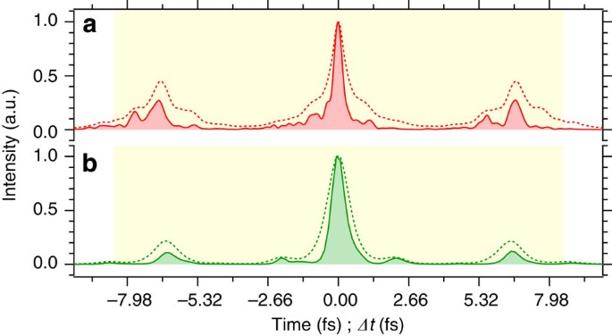Figure 6: Averaged temporal profiles and their AC traces in TC-HHG. (a) Mid-plateau of TC-HH; (b) cutoff of TC-HH. The filled curves and dashed curves exhibit the averaged temporal profiles and their AC traces, respectively. The yellow highlighted region shows the time interval measured in the experiment. Figure 6: Averaged temporal profiles and their AC traces in TC-HHG. ( a ) Mid-plateau of TC-HH; ( b ) cutoff of TC-HH. The filled curves and dashed curves exhibit the averaged temporal profiles and their AC traces, respectively. The yellow highlighted region shows the time interval measured in the experiment. Full size image In addition, we discuss in detail how these pre- and post- pulses at ±6.7 fs affect the measured temporal profiles with the statistical fluctuations of these phases. Here we do not consider the background pedestal under the central main pulse (in the region within ±2.7 fs) originating from weak multiple burst emissions. In Fig. 4b , the peak intensity of the main pulse, the pre- pulse and the post-pulse are plotted versus 0 as blue solid, red dotted and red solid curves, respectively. We can see that the peak intensity of the main pulse reaches its maximum height at a relative phase of 0.14 π , and the pre- and post-pulses are most effectively suppressed at this symmetrical point with peak heights of both 0.08. We find that the highest peak of the pre- and post- pulses in the ± σ region around 0 is lower than 1/ e 2 ~0.14, whereas the area of the normal distribution in our 0 range, which accounts for 68.3% of all events, is depicted as grey-filled area in Fig. 4b . In the second-order AC experiment, the AC intensity of main pulse ( I AC−main ) and the side pulse ( I AC−side ) are given by the square of the main pulse of the CEP-averaged temporal profile ( ) and I main ( I pre + I post ), respectively. Our simulation shows that the event rate of the ± σ region, which has weak pre/post pulse in Fig. 4b , contributes ~85% to the whole AC trace. From this evaluation, we can conclude that the AC signal at the foot of our relative phase distribution (outside the ± σ region) is negligible for composing the AC trace. In other words, the two-photon nonlinear process automatically picks up the most intense IAP part for specific combinations of the CEP and relative phase. As our method has the advantage that the HH output yield can be linearly scaled up by increasing the HH emission volume, we now discuss a scaled-up configuration in the soft-X-ray region to obtain even shorter IAP durations. In the soft-X-ray region at around 100 eV, we have already demonstrated an ~30 nJ energy per harmonic order from OC-HH in Ne gas [22] . By straightforwardly upgrading the TC-HHG to a main pump energy of 50 mJ (with ξ =0.15) and adopting a focusing length of 5 m with a 5-cm-long Ne medium, we can expect to achieve HH pulse energies >0.1 μJ from 95 to 110 eV, which is almost 1,000-fold higher than the energies previously reported [11] . Our simulations indicate that IAPs can be generated with sub-300 as duration. In addition, a straightforward upscaling of the IAP power to a few tens of gigawatts is feasible by extending the focusing length to 50 m with a 100-mJ main pump energy (with ξ =0.15), while maintaining a pulse duration of 500 as at ~30 eV. Since the first demonstration of an IAP was reported in 2001 (ref. 1 ), continuous effort to increase the IAP energy [12] has been exerted by many research groups around the world over the past decade, as illustrated in Fig. 7 . Unfortunately, the output energy of IAPs has not exceeded the nanojoule level thus far. Owing to the low photon flux, the temporal characterization of the IAP was generally achieved using the attosecond streaking method employing frequency-resolved optical gating for complete reconstruction of attosecond bursts (FROG-CRAB) reconstruction. We have now improved the available IAP energy for nonlinear optics experiments by two orders of magnitude compared with the highest output energy reported previously [23] . Our method features good energy scalability and high conversion efficiency owing to the phase-matching technique. We directly characterized the temporal profile of our IAP by an AC method using the nonlinear interaction of N 2 . In fact, the AC traces clearly demonstrate that our HH source is capable of not only inducing nonlinear phenomena but also having attosecond temporal resolution. This experiment also demonstrates the capability of our technique to observe nonlinear attosecond dynamics in real time with IAPs by time-resolved spectroscopy employing a non-sequential two-XUV-photon process in a molecule. Moreover, our intense IAPs are useful as the external injector for a seeded FEL [10] in the XUV region. By combining our attosecond technology and seeded FEL technology, we might obtain an altogether novel XUV light source in the near future. In addition, the quasi-IAP from the mid-plateau of TC-HH will be useful for several applications, for example, for the control of electron localization [24] by attosecond pulse trains, the manipulation of the HHG process [25] , [26] and pump–probe experiments involving a few-cycle laser pulse. Now, the IAP energy has reached the microjoule level, which is 10,000 times higher than the energy of the first demonstration. We think that the presented method paves the way for the intense attosecond science frontier, which will certainly bring a great leap forward in research on ultrafast phenomena and nonlinear optics. 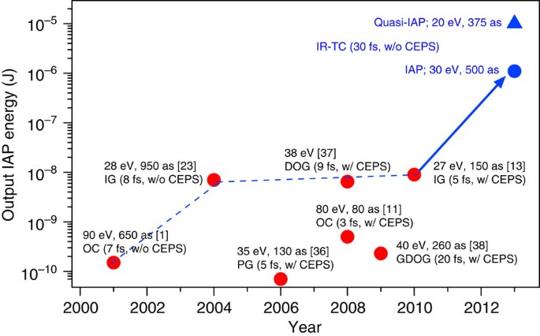Figure 7: Progress of the energy of IAPs used in attosecond experiments. Red circles: previous milestone results using various schemes; blue points: our HHG source. IG, ionization gating; PG, polarization gating; DOG, double optical gating; GDOG, generalized DOG. We indicate the required laser pulse duration and CEP stabilization (CEPS) for each generation scheme. Note the dramatic leap in IAP energy, which is used in an attosecond experiment, by two orders of magnitude achieved in this work. Figure 7: Progress of the energy of IAPs used in attosecond experiments. Red circles: previous milestone results using various schemes; blue points: our HHG source. IG, ionization gating; PG, polarization gating; DOG, double optical gating; GDOG, generalized DOG. We indicate the required laser pulse duration and CEP stabilization (CEPS) for each generation scheme. Note the dramatic leap in IAP energy, which is used in an attosecond experiment, by two orders of magnitude achieved in this work. Full size image Generation configuration for intense attosecond pulses From the point of view of energy scaling for IAPs, the following essential factors have to be considered: (i) scalability of the pump laser energy, (ii) high conversion efficiency of the HHG and (iii) scalability of the generation geometry of HHG. As proposed and demonstrated in ref. 14 , our infrared-TC scheme enables us not only to relax the requirements for the pump pulse duration (~30 fs) and the CEP stabilization but also to markedly minimize the ionization of the harmonic medium. This is a major advantage for efficiently generating intense attosecond pulses, because neutral media allow us to use the phase-matching technique. We strictly considered and designed the configuration of our infrared-TC scheme for scaling up the HH output energy. The supplemental infrared wavelength is optimized to 1,300 nm to effectively suppress satellite pulses on both sides of the central pulse. To extract the HH energy efficiently, the harmonic medium should be extended to satisfy the absorption-limited condition [15] under the phase-matching condition. In the infrared-TC scheme, the difference in group delay between the 800-nm ( λ 0 ) and 1,300-nm ( λ 1 ) pulses even in Xe gas is evaluated to be just 9 as in the 12-cm-long medium of Xe (1 Torr). As this amount is negligible for the synthesized TC field, we can perfectly maintain the waveform in the harmonic medium during propagation. Next, to achieve the highest possible conversion efficiency of HHG in the infrared-TC scheme, we study the effect of ξ (= I IR / I 800nm ) on the conversion efficiency by numerical simulations. The HH yield generally decreases with increasing driving wavelength, which is proportional to λ −α with 5≤ α ≤6 (ref. 27 ). To investigate the scaling exponent α in the TC-HHG, we computed the HH yield by solving the time-dependent Schrödinger equation (TDSE), where V ( r ) is the atomic potential and atomic units are used. We assume that the laser pulse is polarized along the z direction. The TDSE is solved in spherical coordinates, so z = r cos θ . We consider a hydrogen target and V ( r )=−1/ r . The linearly polarized electric field is expressed by where K is the frequency ratio between the main field ( ω 0 ) and the supplemental infrared field ( K = ω 0 / ω 1 , K >1). The subscripts 0 and 1 denote the main fundamental laser and supplemental infrared pulse, respectively. E is the electric field; τ 0,1 , CE and 0 denote the pulse durations, CEP and relative phase, respectively. Note that the jitter in temporal delay δt 1 and in relative phase 0 introduced by path-length fluctuations of the interferometer are connected via δt 1 = K 0 / ω 0 . Here the pulse durations of the fundamental and infrared pulses are both 30 fs, and the total peak intensity is kept constant at I TC =6 × 10 13 W cm −2 . To determine α for each ξ , the central wavelength of the main pulse is kept at 800 nm and that of the infrared pulse is varied from 900 nm to 2,500 nm. ξ is varied from 0 to ∞, the two limits corresponding to OC-HH with λ 0 and OC-HH with λ 1 , respectively. The TDSE is solved using the method described in ref. 28 . The results shown in the inset of Fig. 8 indicate that the scaling exponent α rapidly increases when increasing the relative intensity ξ and finally approaches ~5.5. A high ξ is disadvantageous for the conversion efficiency, even if a good suppression of the shoulder pulses on both sides of the central pulse as well as an extension of the HH cutoff can be obtained. We investigated an upper limit of ξ , for which both a relatively high conversion efficiency and a good suppression of shoulder pulses are simultaneously realized, and we decided to use ξ ~0.15. For ξ =0.15, we find that the HH yield obeys a scaling law of ~ K −0.7 with the wavelength ratio K = λ 1 / λ 0 (see Fig. 8 ). Moreover, we emphasize that our infrared-TC method can universally be applied while maintaining the energy-scaling strategy of HHG, independent of the harmonic medium. 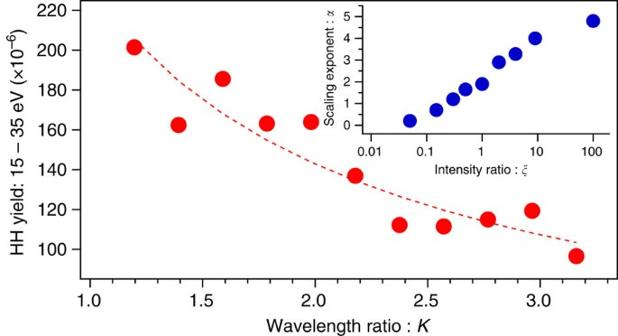Figure 8: HH yield as a function of the wavelength ratioK=λ1/λ0. The relative intensity ratioξ=IIR/I800nmis fixed to be 0.15. Dashed line:α=0.7 scaling. Inset: scaling exponentα(from HH yieldK−α) as a function ofξ. Figure 8: HH yield as a function of the wavelength ratio K = λ 1 / λ 0 . The relative intensity ratio ξ = I IR / I 800nm is fixed to be 0.15. Dashed line: α =0.7 scaling. Inset: scaling exponent α (from HH yield K − α ) as a function of ξ . Full size image Experimental setup 800-nm and infrared pulses are generated starting from a homebuilt TW-Ti:sapphire laser system (30 fs, 150 mJ, 800 nm, 10 Hz; Fig. 9 ). Infrared pulses with a 40-fs duration are produced by a white-light-seeded high-energy optical parametric amplifier [29] . To correct for the different focal lengths of the 800-nm and infrared pulses, both pulses were focused using two separate focusing lenses ( f =4.5 m for 800 nm, f =3.5 m for infrared). We discuss the stability of the interferometer part to produce the TC field in the Discussion section. The two beams are collinearly combined with a dichroic beam splitter and delivered into the target chamber through a thin CaF 2 window. The focused beams pass through the interaction gas cell, which has two pinholes on the entrance and exit surfaces for maintaining the vacuum. The confocal parameters of the two beams are adjusted to be the same, matching the Gouy phase shift through the focus. The Xe target gas was statically filled into the interaction cell of 12 cm length. The HH signals were observed with a flat-field normal-incidence XUV spectrometer with a microchannel plate. A charge-coupled device camera detected the two-dimensional fluorescence from a phosphor screen placed behind the microchannel plate. 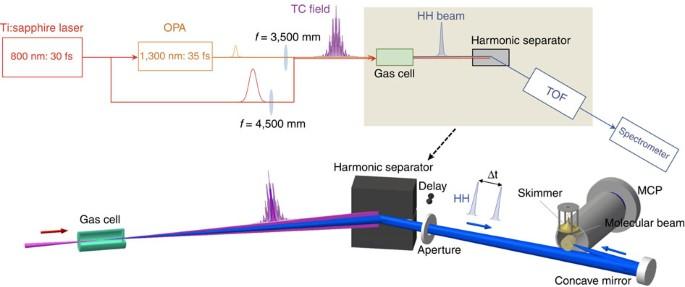Figure 9: Schematic figure of the HHG setup and the second-order autocorrelator. The AC setup (bottom part) is composed of a pair of Si harmonic separators and controls the delay (Δt) between the two replicas of the reflected pulse. The two replica pulses with Δtdelay time are focused by a concave mirror (SiC bulk or Sc/Si multilayer) onto a molecular beam of N2. The fragment ions from N2molecules, which are introduced through a skimmer from a pulsed gas jet, are detected by a TOF ion mass spectrograph, which is constructed from three electrodes, a flight tube, and a microchannel plate (MCP). Figure 9: Schematic figure of the HHG setup and the second-order autocorrelator. The AC setup (bottom part) is composed of a pair of Si harmonic separators and controls the delay (Δ t ) between the two replicas of the reflected pulse. The two replica pulses with Δ t delay time are focused by a concave mirror (SiC bulk or Sc/Si multilayer) onto a molecular beam of N 2 . The fragment ions from N 2 molecules, which are introduced through a skimmer from a pulsed gas jet, are detected by a TOF ion mass spectrograph, which is constructed from three electrodes, a flight tube, and a microchannel plate (MCP). Full size image To evaluate the HH output energy, we first directly measured the total pulse energy of OC-HH from 11th to 21st HH by using an XUV photodiode. The values of spectral sensitivity and quantum efficiency of the XUV photodiode were obtained from ref. 30 and were calibrated with 266-nm Q-switched YAG laser pulses in this experiment. To perfectly block the pump pulse and lower harmonic components (<11th), we inserted a 200-nm-thick Al filter supported by a mesh-back in front of the photodiode. Although the filter transmission of Al can be estimated from the absorption coefficient, the Al filter transmission degrades with time because of oxidation [31] . Therefore, the filter transmission for individual harmonics was calibrated using an XUV spectrometer. From the HH spectral distribution measured by the XUV spectrometer, we divided the total pulse energy among the six harmonic components. Thus, for OC-HH we obtain the relationship between the HH spectral intensity and the pulse energy. In our TC-HH experiments, we computed the area under the measured continuum spectrum by integration within a certain energy range, to evaluate the pulse energy in the cutoff region. When we evaluate the conversion efficiency of HH in the TC-HH case, we used the total pump energy (800 nm+1,300 nm). Indicator of the AC measurement We have adopted the N + ion yield from fragmenting N 2 molecules as the indicator of the second-order AC signal. We show a typical time-of-flight (TOF) mass spectrum of ions at a mass number m/z =14 for irradiation with the mid-plateau TC-HH field in the inset of the bottom panel of Fig. 2a . We can expect that the ion yields in the TOF spectrum contain the N + fragment ions from the dissociative state of N (ref. 32 ) and the Coulomb explosion of N , in addition to doubly charged nitrogen molecular ions N (ref. 33 ) and/or N + ejected through the decomposition pathway of N having zero kinetic energy (KE). The AC function was measured by recording the side-peak yield at KE ~3 eV indicated by the inverted triangle (left side) as a function of the delay time Δ t . The photon energy required for creating these KE peaks around 3 eV is expected to be 32 eV or higher, as deduced from high-resolution coincidence measurements of electrons and N + ions [32] . From the reflectivity of our SiC mirror we conclude that in our situation, the dominant contribution to create the side-peak signals at KE ~3 eV comes from non-sequential two-photon ionization of HH with energies from 12 to 21 eV. When we replaced the focusing mirror from SiC to Sc/Si, we observed the other KE peak of N + at ~5 eV in the TOF spectrum excited by the HH cutoff. We adopted this ion yield as the indicator of the AC signal for the cutoff HH (~30 eV), because a higher KE is expected to contain the signal from Coulomb explosion of N → N + +N + (ref. 34 ) via a two-photon double ionization driven by the cutoff HH. As we could also measure the attosecond pulse train structure when the OC-HH cutoff was employed, we can conclude that the side-peak signal at 5 eV originates from a nonlinear interaction of the HH fields with the N 2 molecules. As is shown in Figs 2 and 3 , the appearance of the AC signal itself in the TOF mass spectra unambiguously proves that there is a nonlinear interaction of HH fields resulting in the production of N + ions at each KE, as a linear interaction cannot provide a correlated signal of the pulse envelope. To discuss the detection sensitivity of our AC measurements, we evaluated the noise-to-peak intensity ratio of the AC trace. Here we defined this ratio according to the following procedure. First, we fit the experimental data points in the middle-bottom panel of Fig. 3 to a Gaussian function. We determined the amplitude of the AC peak ( V amp ) by the fit Gaussian function trace. Next, we subtract the fit Gaussian function trace from the experimental data and evaluated the s.d. ( V sdev ) as the background signal. The signal fluctuations are caused by fluctuations of the measured N + ion yield. The noise-to-peak intensity ratio is defined by V sdev / V amp , resulting in 0.24. Note that we have also evaluated V sdev by simply picking up data points in the ranges outside the correlation peak, which are (−1.15 fs, −0.85 fs) and (0.85 fs, 1.15 fs); again we obtained V sdev / V amp to be 0.21. Thus, we conclude that we can notice side-peak signals with amplitude higher than 0.24 times the main peak height in our AC measurements. Note that the signal-to-background ratio of all our (volume-integrated) second-order AC traces is lower than expected from the theory of the volume-integrated second-order AC. This lower ratio has the same origin as in our past attosecond pulse train measurement, namely the contribution of the single-photon ionization to the background [35] . How to cite this article: Takahashi, E. J. et al. Attosecond nonlinear optics using gigawatt-scale isolated attosecond pulses. Nat. Commun. 4:2691 doi: 10.1038/ncomms3691 (2013).